Resonant Raman spectroscopy of twisted multilayer graphene Graphene and other two-dimensional crystals can be combined to form various hybrids and heterostructures, creating materials on demand with properties determined by the interlayer interaction. This is the case even for a single material, where multilayer stacks with different relative orientation have different optical and electronic properties. Probing and understanding the interface coupling is thus of primary importance for fundamental science and applications. Here we study twisted multilayer graphene flakes with multi-wavelength Raman spectroscopy. We find a significant intensity enhancement of the interlayer coupling modes (C peaks) due to resonance with new optically allowed electronic transitions, determined by the relative orientation of the layers. The interlayer coupling results in a Davydov splitting of the C peak in systems consisting of two equivalent graphene multilayers. This allows us to directly quantify the interlayer interaction, which is much smaller compared with Bernal-stacked interfaces. This paves the way to the use of Raman spectroscopy to uncover the interface coupling of two-dimensional hybrids and heterostructures. Bulk graphite consists of individual graphene planes stacked in a hexagonal (Bernal) [1] structure, or, less commonly, in a rhombohedral [2] one. Single (SLG) or multi-layers (MLG) of graphene can be extracted from graphite by micro-mechanical cleavage [3] . MLGs produced by micro-mechanical cleavage retain the stacking structure of the bulk [4] . The optical and electronic properties of hexagonal or rhombohedral MLGs have significant differences, as shown, for example, in ref. 5 for Bernal and rhombohedral trilayer graphene (TLG). Furthermore, for a given stacking, the band structure significantly changes as a function of the number of layers, N (ref. 6 ). An even wider range of properties is accessible by creating MLG with stacking arrangements different from those common in natural graphite. We refer to these as twisted MLG (tMLG), to indicate a mutual orientation of the planes different from the naturally occurring one. In twisted BLGs, novel physical properties arise because of the periodically modulated interaction between the two Dirac electron gases with a large moiré supercell [7] . These have a Dirac-like linear dispersion with Fermi velocity lower than in SLG [7] , [8] , [9] . By changing the twist angle ( θ t ), it is possible to tune the optical absorption [10] . Twisted BLGs have parallel electronic bands across the Fermi level and the energy of the corresponding van Hove singularities (VHSs) depends on θ t (ref. 11 ). By assembling m -layer ( m LG, m ≥1) and n -layer ( n LG, n ≥1) flakes, a ( m + n )-system is formed, which we indicate as t( m + n )LG. In this notation, a Bernal-stacked BLG is denoted as 2LG, whereas a twisted one as t(1+1)LG. A flake consisting of a Bernal-stacked BLG placed at a generic angle θ t on a Bernal-stacked TLG is indicated as t(2+3)LG. This has significantly different properties when compared with a Bernal-stacked 5LG, or to a t(1+4)LG, or t(1+1+3)LG and so on, even though all these have the same N =5. For a given total N , the choice of m , n and so on (with m + n +...= N ) and relative angles between each m , n ,...LGs leads to a family of systems with different optical and electronic properties [12] , [13] . The ability to probe the interlayer coupling between the interface layers of m LG and n LG in t( m + n )LGs, and its impact on the electronic band structure and lattice dynamics, is crucial to reach a fundamental understanding of these systems and to tune them for novel applications. Raman spectroscopy is one of the most used characterization techniques in carbon science and technology [14] , [15] . The Raman spectrum of graphite and MLG consists of two fundamentally different sets of peaks. Those, such as D, G and 2D, present also in SLG, and due to in-plane vibrations [14] , [16] , [17] , and others, such as the shear (C) modes [18] and the layer breathing modes [19] , [20] , [21] , due to the relative motions of the planes themselves, either perpendicular or parallel to their normal. The G peak corresponds to the high-frequency E 2 g phonon at Γ. The D peak is due to the breathing modes of six-atom rings and requires a defect for its activation [16] , [22] , [23] , [24] . It comes from TO phonons around the Brillouin Zone (BZ) edge K [16] , [22] , is active by double resonance (DR) [24] , and is strongly dispersive with excitation energy due to a Kohn Anomaly (KA) at K [43] . DR can also happen as intra-valley process, i.e. connecting two points belonging to the same cone around K or K ′. This gives the so-called D′ peak. The 2D peak is the D peak overtone. The 2D′ peak is the D′ overtone. Since 2D and 2D′ originate from a process where momentum conservation is satisfied by two phonons with opposite wavevectors, no defects are required for their activation, and are thus always present [4] . In graphite and BLG, there is only one low-frequency E 2 g mode, called C, as it is sensitive to the interlayer coupling [18] . In a MLG comprising N layers, there are N -1 C modes, which we indicate as C NN − i , with i =1..., N −1. In this notation, for a given N , the label C N 1 is used for the highest frequency C peak, which is the only C mode thus far observed in Bernal-stacked MLG [18] . Thus, a TLG has two C modes, C 32 and C 31 , the latter being the highest frequency one. Some of these are Raman active, others are infrared active and others are both, according to symmetry and N (ref. 18 ). The C peak position, Pos(C), is below the notch and edge filter cut of many spectrometers, particularly those suitable for production-line quality monitoring. This problem was overcome by combining BragGrate filters with a single monochromator [18] . This allowed us to measure the highest energy C modes for Bernal-stacked MLGs [18] . However, their intensity, I (C), is much smaller than that of the G peak, I (G), because of the much lower electron-phonon-coupling (EPC) [18] , and it is smaller the lower the Pos(C), for a given N . Thus, so far, the lower energy C modes for a given N could not be detected [18] . Similar C modes exist in any other layered material [18] , [25] , but their intensity is comparable to that of the main high-frequency Raman peaks, allowing for the detection of some of the possible N -1 C modes for a given N [25] , [26] , not just the highest energy one. Note that, albeit being an overtone of an in-plane mode, the 2D peak is sensitive to N since the resonant Raman mechanism that gives rise to it is closely linked to the details of the band structure [4] , [15] , [17] , the latter changing with N , and the layers relative orientation [15] . On the other hand, the C modes are a direct probe of N (ref. 18 ), since the vibrations themselves involve the relative motion of different graphene planes, and not just the relative motion of carbon atoms in a given plane of graphene. Here we study the C modes of t( m + n )LGs. We find that their intensities are enhanced in an excitation energy range depending on m , n and θ t . For a given N = m + n , this allows us to detect m + n −2 C modes arising from the m −1 and n −1 expected for the constituent m LG and n LG in the t( m + n )LG stack. By analysing their Pos(C), we find that the coupling between the graphene layers at the twisted interface can be significantly weaker than that in Bernal-stacked FLGs. The coupling to the layers adjacent to the interface is also softened. In the case of a t(2+2)LG, the out-of-phase and in-phase vibrations of the two twisted, equivalent BLGs, result in a Davydov splitting of ~2 cm −1 for the C peaks of the two constituent BLG peaks. The Raman intensity of the C and G modes is significantly enhanced in t( m + n )LGs for specific excitation energies. This behaviour is assigned to the resonance between VHSs in the joint density of states (JDOSs) of all optically allowed transitions in twisted multilayer samples and the laser excitation energy, during the optical absorption and emission steps of the Raman process. The VHSs contribute to different extent to the resonant profiles, which is a sign of varying EPC for different C bands. Raman spectroscopy of t( n + m )LG We consider a flake comprising SLG, TLG, t(1+1)LG and t(1+3)LG regions, the latter formed by folding SLG onto TLG/SLG during mechanical exfoliation of graphite (see Fig. 1a ; see Methods for details). The optical contrasts of t(1+1)LG and t(1+3)LG in Fig. 1b are, respectively, different from those of 2LG and 4LG. We note that an additional feature appears at ~2 eV for both t(1+1)LG and t(1+3)LG, a fingerprint of the different band structure in twisted samples, when compared with Bernal-stacked ones [27] , [28] . 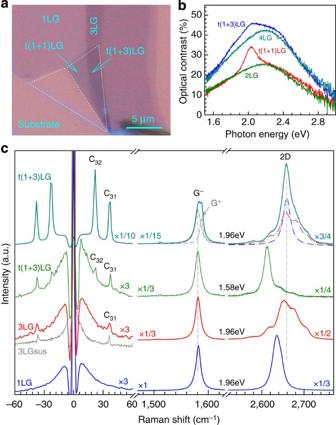Figure 1: Optical characterization and Raman spectra of t(1+3)LG. (a) Optical image of a flake comprising a t(1+1)LG and a t(1+3)LG. (b) Optical contrast of t(1+1)LG and t(1+3)LG. For comparison, the contrast of 2LG and 4LG is also plotted. (c) Stokes/anti-Stokes Raman spectra of 1LG, 3LG and t(1+3)LG on SiO2in the C peak spectral region, and Stokes Raman spectra of 1LG, 3LG and t(1+3)LG in the G and 2D peak spectral regions, for 1.96 eV excitation. 1.58 eV excitation is also used for t(1+3)LG. The C mode of a suspended 3LG (3LGsus) is shown in grey for comparison. The t(1+3)LG 2D band is fitted by the 1LG- and 3LG-like 2D components, as shown with dash–dotted lines, respectively. Figure 1: Optical characterization and Raman spectra of t(1+3)LG. ( a ) Optical image of a flake comprising a t(1+1)LG and a t(1+3)LG. ( b ) Optical contrast of t(1+1)LG and t(1+3)LG. For comparison, the contrast of 2LG and 4LG is also plotted. ( c ) Stokes/anti-Stokes Raman spectra of 1LG, 3LG and t(1+3)LG on SiO 2 in the C peak spectral region, and Stokes Raman spectra of 1LG, 3LG and t(1+3)LG in the G and 2D peak spectral regions, for 1.96 eV excitation. 1.58 eV excitation is also used for t(1+3)LG. The C mode of a suspended 3LG (3LG sus ) is shown in grey for comparison. The t(1+3)LG 2D band is fitted by the 1LG- and 3LG-like 2D components, as shown with dash–dotted lines, respectively. Full size image Figure 1c plots the Raman spectra, measured as described in Methods, in the spectral ranges of the C, G and 2D bands, for an excitation energy E ex =1.96 eV. The spectra are normalized to I(G) of the SLG sample. The 2D band of t(1+3)LG can be fitted using the peak profiles of the SLG and TLG 2D bands, as indicated by the dashed-dotted lines in Fig. 1c . The fitted SLG-like and TLG-like sub-peaks for t(1+3)LG are blue-shifted by ~24 and 5 cm −1 , respectively, relative to those found in pristine SLG and TLG. Note that the full width at half maximum of the G peak, FWHM(G), and Pos(G) of t(1+3)LG measured for 1.58 eV excitation are identical to those of 3LG and 1LG, as indicated in Fig. 1c . Thus, we assume that doping or strain are not responsible for the blue-shift of the 2D bands in t(1+3)LG. The blueshift can be attributed to the decrease of Fermi velocity in t(1+3)LG, similar to what previously reported for t(1+1)LG in refs 7 , 9 , 29 . This is another indication that the constituent SLG and TLG couple with each other in the t(1+3)LG sample, producing a unique band structure, different from that of the individual constituents and from that expected for 4LG. I(G) of t(1+3)LG is also 15 times stronger than that of SLG. As the Raman intensity scales with volume, one would expect I(G) for a sample with 4 layers of graphene to be 4 times bigger than that of a SLG, instead of the 15 times measured here. This suggests a resonant enhancement of I(G) at 1.96 eV. A similar enhancement was previously observed in t(1+1)LG [27] , [29] , where the measured I(G) was 20–60 times bigger than in SLG for a specific excitation energy, instead of the expected factor 2. We also note that FWHM(G) of our t(1+3)LG is ~18 cm −1 , broader than the ~12 cm −1 intrinsic in pristine SLG [30] , [31] . Closer inspection shows that the G band consists of two sub-bands, which we call G − and G + , using a similar terminology to that used in strained graphene [32] . However, the G peak of t(1+3)LG measured at 1.58 eV has a single Lorentzian lineshape, with identical width and position to the G − peak of t(1+3)LG measured at 1.9 eV. This implies that the doubling of the G peak is connected to a resonant process. Figure 1c also shows that the C mode of the SiO 2 -supported 3LG is observed at ~37 cm −1 , with a worse signal-to-noise ratio than that of the suspended 3LG (3LG sus ), because of the strong background from the Si substrate [18] . The t(1+3)LG sample consists of 4 graphene layers. In Bernal-stacked 4LG, 4−1=3 C modes are expected at ~41 (Raman active), 31 (infrared active) and 17 cm −1 (Raman active) [18] , but only one of them at ~41 cm −1 was previously measured [18] . In a TLG, 3−1=2 C modes are expected at ~38 (Raman and infrared active) and 23 cm −1 (Raman active) [18] , but only one of them at ~38 cm −1 was previously measured [18] . In our t(1+3)LG, we detect two C peaks at ~22 and ~37 cm −1 , as confirmed by the presence of their anti-Stokes components. Their positions are in excellent agreement with those expected for the two Raman active modes in TLG, and not with those expected in a 4LG. We thus ascribe them to the C 32 and C 31 of the 3LG constituent in t(1+3)LG, since, of course, SLG cannot have any C mode. We also note that I(C 32 )~I(C 31 )~I(G) in the t(1+3)LG, whereas I(C 31 )/I(G) ~0.02 in TLG, thus the C modes in t(1+3)LG are enhanced a factor ~50. This is another indication that the coupling between the SLG and TLG constituents of the twisted sample results in a heterostructure with properties, such as the band structure, distinct from those of its constituents. Similar results are found for other t( m + n )LGs (see Supplementary Fig. 1 for optical images). 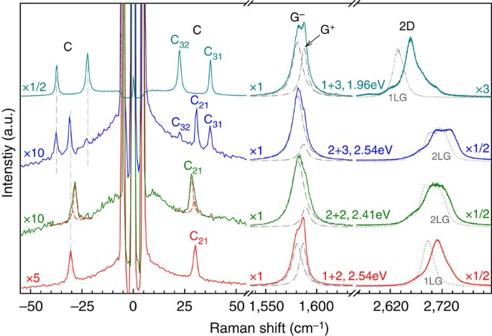Figure 2: Raman spectroscopy of t(m+n)LG. Stokes/anti-Stokes Raman spectra in the C peak region and Stokes spectra in the G and 2D spectral regions for four t(m+n)LGs. For comparison, the 2D peaks in SLG and Bernal-stacked BLG are plotted using dotted lines. The fits show that the G band of each t(m+n)LG is composed of two subpeaks, G−and G+. The excitation energy used for each t(m+n)LG is indicated. The spectra are scaled and offset for clarity. The scaling factors of the individual spectra are also shown. Figure 2 shows the Stokes (S) and anti-Stokes (AS) spectra in the C spectral region and Stokes spectra in the G and 2D spectral regions for four t( m + n )LGs with m =1 or 2 and n =2 or 3. To facilitate comparison, all spectra are normalized to their respective I(G). The 2D bands of all t( m + n )LGs are blue-shifted relative to those measured under the same conditions for SLG, BLG, TLG, as also seen in Fig. 1 . In the t(1+2)LG sample, we detect only one C mode located at ~30 cm −1 , close to Pos(C BLG )=32 cm −1 measured for Bernal-stacked BLG [18] . t(2+2)LG exhibits a broad and asymmetrical peak with FWHM=2.2 cm −1 , once the system resolution (~0.5 cm −1 ) is accounted for. This is 1.2 cm −1 bigger than that (~1 cm −1 ) measured in Bernal-stacked BLG. In fact, this band can be fitted using two Lorentzians at ~28.9 cm −1 and 30.6 cm −1 , denoted as C 21 − and C 21 + , respectively. In t(2+3)LG, besides the two C modes of its 3LG constituent, an additional mode at 30.8 cm −1 related to its 2LG constituent is present, with a small FWHM ~1 cm −1 . In t(1+3)LG, as shown in Fig. 1 and discussed above, two C modes related to its 3LG constituent are observed. In short, m + n −2 C modes are observed in a t( m + n )LG for specific excitation energies, instead of m + n −1 C modes expected in Bernal-stacked ( m + n )LGs. The observed modes are related to the C modes of the constituent m LG (if m >1) and n LG ( n >1). The frequencies of all C modes shown in Fig. 2 are summarized in Fig. 3a using open diamonds. Figure 2: Raman spectroscopy of t( m + n )LG. Stokes/anti-Stokes Raman spectra in the C peak region and Stokes spectra in the G and 2D spectral regions for four t( m + n )LGs. For comparison, the 2D peaks in SLG and Bernal-stacked BLG are plotted using dotted lines. The fits show that the G band of each t( m + n )LG is composed of two subpeaks, G − and G + . The excitation energy used for each t( m + n )LG is indicated. The spectra are scaled and offset for clarity. The scaling factors of the individual spectra are also shown. 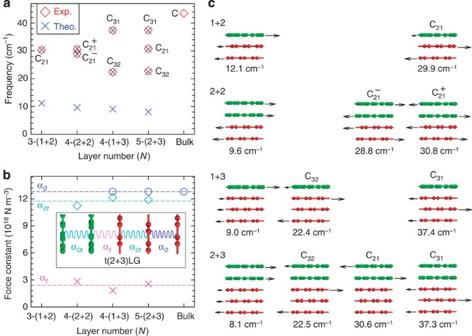Figure 3: Shear mode frequencies and normal mode displacements in t(m+n)LG. (a) Experimental (Exp., open diamonds) and theoretical (Theo., crosses) Pos(CNN−i) in t(m+n)LGs (N=m+n). (b) Fitted shear force constants (αtandα0t) in t(m+n)LGs. The inset shows a schematic diagram of a linear chain model for t(2+3)LG including a bulk interlayer force constant,α0, interface force constant,αtand the softened force constant for the layers adjacent to the interface,α0t. (c) Normal mode displacements and mode frequencies from the linear chain model inb. Full size image Figure 3: Shear mode frequencies and normal mode displacements in t( m + n )LG. ( a ) Experimental (Exp., open diamonds) and theoretical (Theo., crosses) Pos(C NN − i ) in t( m + n )LGs ( N = m + n ). ( b ) Fitted shear force constants ( α t and α 0 t ) in t( m + n )LGs. The inset shows a schematic diagram of a linear chain model for t(2+3)LG including a bulk interlayer force constant, α 0 , interface force constant, α t and the softened force constant for the layers adjacent to the interface, α 0t . ( c ) Normal mode displacements and mode frequencies from the linear chain model in b . Full size image Similar to t(1+3)LG, a G − and G + double peak structure is observed in the G peak region for all t( m + n )LGs, as revealed by the Lorentzian fits shown in Fig. 2 . Also, for each t( m + n )LG, the G + mode can only be observed in a small E ex range (see the Supplementary Fig. 2 ), whereas the G − component always exists. The G + peak is observed neither in Bernal-stacked SLG, TLG, 4LG nor in t(1+1)LG. The observed G + position in t( m + n )LGs is 6–7 cm −1 higher than the G peak in a Bernal-stacked N (= m + n )LG, whereas the G − component is at ~1,581 cm −1 , independent on E ex . We note that the split between the Raman-active and infrared-active E 1 u modes in bulk graphite is ~6 cm −1 (ref. 33 ). Therefore, one might attribute the G + peak in t( m + n )LGs to the E 1 u -like zone-centre mode of their 2LG and 3LG constituents. Interlayer coupling at the twisted interface To understand the interlayer coupling in t( m + n )LG, we use the linear chain model introduced in ref. 18 . However, in the case of twisted samples, we need to consider that the interlayer coupling between the constituent Bernal-stacked sub-layers may not be the same as that inside each Bernal-stacked layer and that the presence of the interface perturbs the force constant between the two layers closest to the interface in both sub-layers. We denote the interlayer shear force constant between two sub-layers ( m LG and n LG) by α t and the perturbed force constant adjacent to the interface in m LG and/or n LG by α 0 t . The force constant per unit area between bulk layers away from the interface is given by α 0 . In FLGs, this interlayer force constant was experimentally determined to be α 0 =12.8 × 10 18 Nm −3 (ref. 18 ). The force constants are illustrated in the inset of Fig. 3b for a t(2+3)LG case. The frequencies ω (in cm −1 ) and displacement patterns of the shear modes in t( m + n )LG can be calculated by solving linear homogeneous equations follows [34] : where u i is the phonon eigenvector of the mode i with frequency ω i , μ =7.6 × 10 −27 kg Å −2 the monolayer mass per unit area, c =3.0 × 10 10 cm s −1 the speed of light and D the shear part of the force constant matrix (for details, see Supplementary Note 1). Based on the experimental C mode frequencies of t(2+2)LG, t(1+3)LG and t(2+3)LG, we can fit the parameters α 0t and α t . The average values for α 0t and α t are 11.8 × 10 18 Nm −3 and 2.4 × 10 18 Nm −3 , respectively. These values suggest that the interlayer coupling at the interface between the twisted Bernal layers is ~5 times weaker than the coupling in the Bernal-stacked layers, whereas the coupling between layers next to the interface, α 0t , decreases by ~9% with respect to α 0 . The theoretical and experimental Pos(C NN − i ) in t( m + n )LGs are summarized in Fig. 3a as crosses and open diamonds, respectively. Figure 3c shows the normal mode displacements calculated using equation (1). The mode displacements are mainly localized within the n LG or m LG constituents and they are only weakly affected by the coupling across the twisted interface. We also note that a low-frequency mode below 15 cm −1 is theoretically predicted. This corresponds to the relative vibration of the m LG and n LG constituents in t( m + n )LGs, as illustrated in Fig. 3c . However, we have not been able to detect this in our experiments to date, possibly due to a very weak EPC. Davydov splitting of the C mode In Fig. 2 , two subpeaks, split by ~2 cm −1 , are found for the t(2+2)LG C peak. It is interesting to compare the lattice dynamics of t(2+2)LG and Bernal-stacked 4LG. The C 41 mode of 4LG at 41 cm −1 does not exist in t(2+2)LG because of the weak coupling at the interface. The C 42 mode at ~31 cm −1 of 4LG is infrared-active [18] . As shown in Fig. 3b in ref. 18 , for this mode the two middle layers move in phase, and the two BLGs are out-of-phase with respect to each other. Thus, the mode displacement is similar to that in two uncoupled BLGs. Thus, Pos(C 42 )~31 cm −1 is equal to that of the C mode in 2LG (the latter, however, corresponding to a Raman active mode) [18] . In t(2+2)LG, the displacements of the middle layers are in-phase for C 21 − . Its lower frequency (28.8 cm −1 ) than that of the BLG C 21 and 4LG C 42 suggests a softening of the coupling between layers next to the interface. C 21 + has a higher frequency than C 21 − because the weakly coupled middle layers vibrate out-of-phase in this case. If this coupling were as strong as in the Bernal-stacked case, Pos(C 21 + ) would be much higher than Pos(C 21 − ), close to Pos(C 41 ) in 4LG. The frequency difference between C 21 − and C 21 + is referred to as Davydov splitting [35] , which is the frequency difference of two conjugate vibration modes. Such splitting is a direct signature of the presence of coupling, albeit weak, between the two interface layers. The weak interlayer coupling at the interface between the constituent BLGs is also confirmed by analysing the positions of the three C modes in t(2+2)LG. The frequency of the relative vibration between the two constituent BLGs in t(2+2)LG can be approximately deduced [36] as , which agrees well with the calculated 9.6 cm −1 . A similar C mode Davydov splitting is expected to occur in all t( n + n )LGs. Raman intensity The C and G + modes for each t( m + n )LG can only be detected in a small E ex range, suggesting a resonant mechanism. Here we consider in detail the case of t(1+3)LG and a reference t(1+1)LG, where no C nor G + peaks are expected. 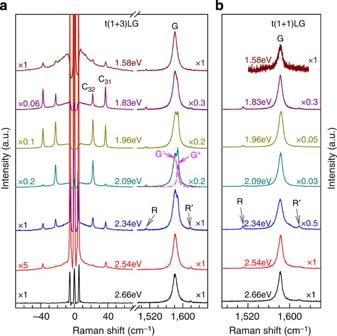Figure 4: Raman spectra of t(1+3)LG and t(1+1)LG at different excitation energies. (a) C and G modes of t(1+3)LG and (b) G mode of t(1+1)LG for sevenEex. The R and R′ modes are indicated by arrows. The presence of theG+mode is revealed by the two-Lorentzian fit to the t(1+3)LG G band measured at 2.09 eV. The spectra are scaled and offset for clarity. The scaling factors of the individual spectra are also shown. Figure 4 plots the measured spectra at seven wavelengths both for t(1+1)LG and t(1+3)LG, with peak intensities normalized to I(G) in a SLG. I(G) in t(1+1)LG and I(C), I(G − ) and I(G + ) in t( 1+3)LG strongly depend on E ex . Figure 4a shows that the G + peak in t(1+3)LG can only observed in a small E ex range. Figure 4: Raman spectra of t(1+3)LG and t(1+1)LG at different excitation energies. ( a ) C and G modes of t(1+3)LG and ( b ) G mode of t(1+1)LG for seven E ex . The R and R′ modes are indicated by arrows. The presence of the G + mode is revealed by the two-Lorentzian fit to the t(1+3)LG G band measured at 2.09 eV. The spectra are scaled and offset for clarity. The scaling factors of the individual spectra are also shown. Full size image In order to explain the origin of the resonant enhancement, we calculate the band structure corresponding to our t(1+1)LG and t(1+3)LG samples. θ t determines the coupling between the constituent n LG and m LG and needs to be known to perform meaningful calculations. θ t can also be expressed in terms of the twist vector [7] , [37] ( p , q ). The so-called R and R′ Raman bands have been suggested as probes of θ t in t(1+1)LG [38] , [39] . As shown in Fig. 1a , in our experiment the same SLG is folded onto both SLG and TLG regions to form the t(1+1)LG and t(1+3)LG samples. Consequently, as the top and bottom layers in our t(1+1)LG and t(1+3)LG are the same SLG, both systems have the same θ t . The R and R′ peaks of our t(1+1)LG are measured to be ~1,510 and 1,618 cm −1 , whereas in the t(1+3)LG, they are at ~1,512 and 1,618 cm −1 . From the position of the R band, θ t can be determined as ~10.6° for both t(1+1)LG and t(1+3)LG, following the procedure used in ref. 39 for a t(1+1)LG sample. This is close to a twist vector of (1,9) and θ t =10.4°. The optical contrast of t(1+1)LG in Fig. 1b shows an absorption peak at ~2.03 eV, which agrees with that calculated in ref. 39 for (1,9) t(1+1)LG. We thus use a twist vector of (1,9) and θ t =10.4° in our band structure calculations for t(1+1)LG and t(1+3)LG. We calculate the band structure of (1,9) t(1+1)LG with the Density Functional based Tight Binding (DFTB+) code, as discussed in Methods [40] , in Fig. 5a . 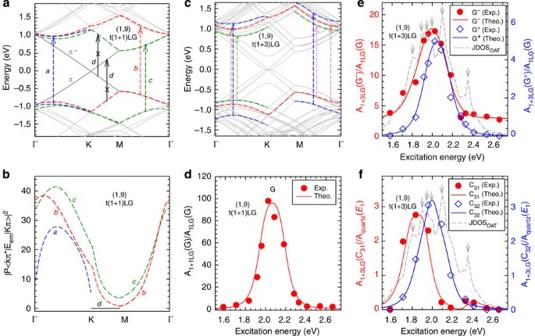Figure 5: Intensity resonance of the C and G modes. (a) Band structure of (1,9) t(1+1)LG. The optically allowed transitions are marked by dashed arrows. The transitions with energy ~1.15 eV between parallel bands alongK-Mare forbidden, as indicated by solid arrows with crosses. (b) Squared optical matrix elements of the corresponding band pairs ina. (c) Band structure of (1,9) t(1+3)LG. Some typical transitions are indicated by vertical dashed lines. (d) A(G) of t(1+1)LG, (e) A(G−) and A(G+) of t(1+3)LG, and (f) A(C31) and A(C32) as a function of laser excitation energy. The filled circles and open diamonds are the experimental data, while the solid lines show the simulations. The grey dash–dotted lines ineandfare the electronic joint density of states (JDOSs) of all the optically allowed transitions (JDOSOAT) in t(1+3)LG along Γ-K-M-Γ. The VHSs of JDOSOATare indicated with arrows. Figure 5b plots the squared optical matrix elements for pairs of electronic transitions between conduction and valence bands in Fig. 5a . The electronic transitions are optically allowed if the corresponding squared optical matrix element is non-zero. For example, the optical transitions of (1,9) t(1+1)LG between two parallel conduction and valence bands along the K - M direction, labelled by the two arrows with crosses in Fig. 5a , are optically forbidden because of their zero squared optical matrix element, as indicated by curve d in Fig. 5b , as the corresponding Raman matrix element expressed within the third-order perturbation theory is quenched. The optically allowed transitions in (1,9) t(1+1)LG are indicated by dashed lines with arrows. The optical matrix elements are anisotropic along the high-symmetry directions, as for Fig. 5b . Figure 5: Intensity resonance of the C and G modes. ( a ) Band structure of (1,9) t(1+1)LG. The optically allowed transitions are marked by dashed arrows. The transitions with energy ~1.15 eV between parallel bands along K - M are forbidden, as indicated by solid arrows with crosses. ( b ) Squared optical matrix elements of the corresponding band pairs in a . ( c ) Band structure of (1,9) t(1+3)LG. Some typical transitions are indicated by vertical dashed lines. ( d ) A(G) of t(1+1)LG, ( e ) A(G − ) and A(G + ) of t(1+3)LG, and ( f ) A(C 31 ) and A(C 32 ) as a function of laser excitation energy. The filled circles and open diamonds are the experimental data, while the solid lines show the simulations. The grey dash–dotted lines in e and f are the electronic joint density of states (JDOSs) of all the optically allowed transitions (JDOS OAT ) in t(1+3)LG along Γ- K - M -Γ. The VHSs of JDOS OAT are indicated with arrows. Full size image The band structure of (1,9) t(1+3)LG is shown in Fig. 5c . In the low-energy region, two parabolic bands from the 3LG can still be seen. A linear band arising from the SLG constituent is superimposed with that of the TLG constituent to form a doubly degenerate linear band, with a Fermi velocity ~4% smaller than in SLG, because of the coupling at the interface. This reduction manifests itself in a blueshift of the SLG-like 2D peak in Fig. 1c . The selection rule for optically allowed transitions in t(1+3)LG is more complex than in t(1+1)LG. As an example, some optically allowed transitions in t(1+3)LG are shown in Fig. 5c with vertical arrows. This results in a broader absorption peak in t(1+3)LG in comparison to t(1+1)LG, as shown in Fig. 1b . The experimental areas of the G band in t(1+1)LG [A(G)] and the G and C bands in t(1+3)LG [A(G − ),A(G + ), A(C 31 ) and A(C 32 )] as a function of E ex are plotted in Fig. 5d–f . The G modes are normalized to A(G) of SLG, whereas the C modes are normalized to the quartz substrate E 1 modes (at 127 cm −1 ) [41] to eliminate the effect of different charge-coupled device (CCD) efficiencies at each E ex . The Raman intensity of the C and G modes is then calculated by second-order perturbation theory [42] . Because only the optically allowed electronic transitions can be involved in the resonant Raman process [27] , we calculate the electronic JDOSs of all the optically allowed transitions (JDOS OAT ) in t( m + n )LG by the following equation: where M ij ( k ) is the optical matrix element between the i th conduction and j th valence bands, E ij ( k ) gives the transition energy of a i → j band pair at the wavevector k , 180 k -points are used for the summation along the Γ- K - M -Γ path, distributed according to the respective path lengths in the reciprocal space. The optically allowed transitions in t(1+1)LG shown in Fig. 5a contribute to a VHS at 1.95 eV with FWHM=0.13 eV (see Supplementary Fig. 3 ). The JDOS OAT for t(1+3)LG is shown in Fig. 5e,f by grey dashed lines. There are six distinctive VHSs in the JDOS OAT of (1,9) t(1+3)LG, which are labelled by arrows (see the Supplementary Fig. 4 ). t(1+3)LG has broader JDOS OAT (FWHM=0.5 eV) than t(1+1)LG, because of its more complex band structure. The major contribution to the intensity comes from resonance matching between E ex and the VHSs energies of the JDOS OAT . Therefore, the intensity of Raman modes in t( m + n )LG as a function of E ex can be evaluated as [39] : where M j are constants treated as fitting parameters that encompass the product of the electron–phonon and electron-photon interactions matrix elements for the j th VHS in the JDOS OAT , E ph is the phonon energy (0.196 eV for G , 0.197 eV for G + , 4.6 meV for C 31 , 2.7 meV for C 32 ) and γ gives the energy uncertainty related to the lifetime of the excited state. Here we assume γ =0.15 eV. The calculated A(C) and A(G) as a function of E ex are shown in Fig. 5d–f with solid curves. Both are in good agreement with experiments. The resonant profile of the G + peak for t(1+3)LG is symmetric and centred at 2.05 eV with a width of 0.3 eV, which indicates that the VHSs of JDOS OAT with lower (<1.8 eV) and higher (>2.3 eV) energies contribute little to it. However, that of the G − peak is asymmetric and slightly broader, implying that the corresponding VHSs with a wider energy range contribute to its resonance, particularly in the lower energy range (<1.9 eV). When out of resonance, the G + peak vanishes, whereas I(G − ) of t(1+3)LG is about three times that of I(G) in SLG. Because of the small energy of the C phonon, the resonance condition for both incoming and outgoing photons can be simultaneously nearly fulfilled. This significantly enhances A( C NN − i ) when in resonance with the optically allowed transitions in t(1+3)LG, as demonstrated in Fig. 5c,f . Indeed, A(C 31 ) and A(C 32 ) excited at 1.96 eV are ~120 and 190 times that of A(C 31 ) in Bernal-stacked 3LG, and are comparable to A(G − ) and A(G + ). In particular, both C 31 and C 32 exhibit broad resonant profiles with a width comparable to that of the G − and G + peaks. The resonant profile of C 32 is blue-shifted by 0.13 eV relative to that of C 31 . A( C 32 ) is resonantly enhanced by the transitions associated with VHSs at 2.1 eV, which contribute little to A( C 31 ), whereas A( C 31 ) is significantly enhanced by the transitions associated with VHSs below 1.8 eV. Note that there is a weak resonant peak at 2.4 eV for A( C 31 ), which corresponds to the VHSs at 2.36 eV. For an electronic transition at some wavevector k , the matrix elements related with electron–photon interactions are the same for C 31 and C 32 . The EPC matrix element, however, can be different. Indeed, the EPC strength greatly varies for the different graphene phonon branches [31] , [42] , [43] . As the EPC of C 41 in 4LG is ~15 times larger than the other Raman-active C 43 mode at 17 cm −1 , the other C modes are challenging to detect [18] . The observation of different resonant profiles for C 31 and C 32 indicates that, in addition to differences in the EPC strength, the EPC is also anisotropic in the k space, thus removing the contribution from some optically allowed transitions to the resonant Raman process of some vibration modes. This results in the significant difference between the resonant profiles of C 31 and C 32 , although their phonon energy is smaller than 5 meV. This also explains the different resonant behaviour of G − and G + . The C mode of Bernal-stacked FLG can be fitted with a Breit-Wagner-Fano (BWF) line shape [18] . This is attributed to quantum interference between the C mode and a continuum of electronic transitions near K (ref. 18 ). Our calculation of the t(1+3)LG band structure reveals that twisting cannot induce a band gap near K . Therefore, a similar BWF profile can be present for the C mode in the twisted system, similar to that in Bernal-stacked 3LG. However, the intensity enhancement of the C mode in t(1+3)LG masks the weak BWF profile, giving an overall Lorentzian profile. The weak coupling between the two interface layers in t( m + n )LGs can be understood considering the nature of C modes, that originate from interlayer shear vibrations. Because of the twist, the atoms at the interface are misaligned with respect to each other, which results in a weaker moiré-modulated coupling between the two interface layers, compared with the ordered arrangement in conventional AA-, AB- or ABC-stacked FLG. Because the C peak positions directly reflect the interlayer interactions, the measurement of the C modes in t( m + n )LG allows the direct evaluation of interlayer interactions, both at the twisted interface and in the neighbouring layers. The coupling across this interface is weaker than the interaction between Bernal-stacked layers. Nevertheless, such a weak interaction can modify the electronic dispersion, as proven by the resonant enhancement of the C modes. This paves the way to the use of Raman spectroscopy to uncover the interface coupling of two-dimensional hybrids and heterostructures. Sample preparation Highly oriented pyrolytic graphite is mechanically exfoliated on a Si substrate covered with a 90-nm SiO 2 to obtain multilayer graphene [44] . To form t( m + n )LG, a m LG flake is folded onto a n LG during the exfoliation process, or a m LG flake from one Si substrate is transferred onto a n LG on another Si substrate. The number of layers in all initial and twisted flakes is identified by Raman spectroscopy and optical contrast [4] , [45] , [46] . Raman measurements Raman spectra are measured in back-scattering at room temperature with a Jobin-Yvon HR800 Raman system, equipped with a liquid-nitrogen-cooled CCD, a × 100 objective lens (numerical aperture=0.90) and several gratings. The excitation energies are 1.58 and 1.71 eV from a Ti:Saphire laser, 1.96, 2.03, 2.09 and 2.28 eV from a He-Ne laser, 1.83, 1.92, 2.18, 2.34 and 2.41 eV from a Kr + laser, and 2.54, 2.67 eV from an Ar + laser. The resolution of the Raman system at 2.41 eV is 0.54 cm −1 per CCD pixel. Plasma lines are removed from the laser signals, using BragGrate Bandpass filters. Measurements down to 5 cm −1 for each excitation are enabled by three BragGrate notch filters with optical density 3 and with FWHM=5–10 cm −1 (ref. 18 ). Both BragGrate bandpass and notch filters are produced by OptiGrate Corp. The typical laser power is ~0.5 mW, to avoid sample heating. Calculations Band structure calculations are carried out using DFTB in its DFTB+ implementation [40] , [47] , [48] . This code is based on a second-order expansion of the Kohn–Sham total energy in Density-Functional Theory [49] , [50] with respect to charge density fluctuations. The Coulomb interaction between partial atomic charges is determined using the self-consistent charge formalism [51] . A Slater Kirkwood-type dispersion [52] is employed for the van der Waals and π – π stacking interactions. Here we adopt the parameter set ‘mio-0-1’ [51] for Slater–Koster files. This approach was shown to give reasonably good prediction of the band structure in graphene and related systems [53] , [54] . To calculate the optical matrix elements, the tight-binding model of refs 7 , 55 is used. The model hopping parameters are scaled by 18% (refs 27 , 29 , 56 ) to compensate for the underestimation of Fermi velocity in the absence of corrections because of electron–electron interactions [57] . The optical matrix elements are calculated as [42] : where denotes the i th state in the valence (conduction) band and P in[out] is the light polarization. Unpolarized light is considered by summing incoherently over x and y polarizations. How to cite this article: Wu, J.-B. et al. Resonant Raman spectroscopy of twisted multilayer graphene. Nat. Commun. 5:5309 doi: 10.1038/ncomms6309 (2014).